Spirocyclic hypervalent iodine(III)-mediated radiofluorination of non-activated and hindered aromatics Fluorine-18 ( t ½ =109.7 min) is the most commonly used isotope to prepare radiopharmaceuticals for molecular imaging by positron emission tomography (PET). Nucleophilic aromatic substitution reactions of suitably activated (electron-deficient) aromatic substrates with no-carrier-added [ 18 F]fluoride ion are routinely carried out in the synthesis of radiotracers in high specific activities. Despite extensive efforts to develop a general 18 F-labelling technique for non-activated arenes there is an urgent and unmet need to achieve this goal. Here we describe an effective solution that relies on the chemistry of spirocyclic hypervalent iodine(III) complexes, which serve as precursors for rapid, one-step regioselective radiofluorination with [ 18 F]fluoride. This methodology proves to be efficient for radiolabelling a diverse range of non-activated functionalized arenes and heteroarenes, including arene substrates bearing electron-donating groups, bulky ortho functionalities, benzylic substituents and meta -substituted electron-withdrawing groups. Polyfunctional molecules and a range of previously elusive 18 F-labelled building blocks, compounds and radiopharmaceuticals are synthesized. Fluorine-18 ( 18 F; t ½ =109.7 min) labelled compounds and radiopharmaceuticals are the mainstay of functional molecular imaging by positron emission tomography (PET) for a broad range of applications including clinical diagnosis and drug discovery [1] , [2] , [3] , [4] , [5] . Consequently, there is a rapidly growing demand for new 18 F-labelled agents to probe biological processes and targets in vivo [6] . Fluorine-18 is most readily prepared in high specific activity as no-carrier-added [ 18 F]fluoride ion, by proton irradiation of [ 18 O]H 2 O ( 18 O(p,n) 18 F nuclear reaction) in medical cyclotrons. Most 18 F-labelling methodologies for nucleophilic aromatic substitution (S N Ar) reactions employ ‘naked’ [ 18 F]fluoride ion with appropriately activated (electron-deficient) aromatic/heteroaromatic substrates. However, radiofluorination of non-activated arenes represents a major challenge in the field and there is an urgent need for a general and practical methodology that can introduce 18 F into molecules that cannot be labelled using a conventional S N Ar reaction. Reactions of non-activated arenes with [ 18 F]fluoride by Balz–Schiemann reactions with diazonium tetrafluoroborate salts [7] or Wallach reactions with triazene-based precursors [8] have proven to be inefficient and low yielding. Other efforts to achieve this goal include applications of triarylsulphonium salts [9] , diarylsulphoxides [10] or the post-S N Ar conversion of activating, electron-withdrawing groups into electron-donating groups, for example, through Baeyer–Villiger oxidation [11] , all of which are based on reactions towards electron-deficient arenes and have limited substrate scope. Alternatively, transition-metal-mediated fluorination reactions ( Fig. 1a, 1 ) [12] , [13] and oxidative fluorination of phenol derivatives [14] ( Fig. 1a, 2 ) have been investigated. Unfortunately, the latter two methods employ air-sensitive complexes of toxic metals ( 1 ) or have yet to demonstrate extensive substrate scope ( 2 ). 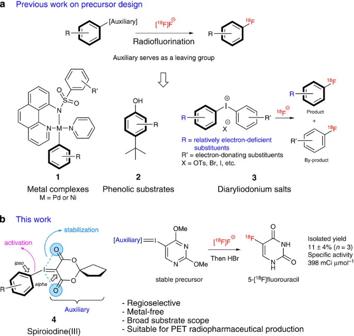Figure 1: Direct radiofluorination of non-activated arenes. (a) Previous work on precursor design. (b) This work. Figure 1: Direct radiofluorination of non-activated arenes. ( a ) Previous work on precursor design. ( b ) This work. Full size image The introduction of [ 18 F]fluoride ion into electron-rich or -deficient arenes via diaryliodonium salt-based precursors ( Fig. 1a, 3 ) [15] , [16] , [17] has been recently reviewed [18] , [19] . This technology has been successfully used to prepare PET radiopharmaceuticals. However, 18 F-incorporation into the relatively electron-deficient (activated) arene is accompanied by production of undesired radioactive byproducts arising from the electron-rich aryl auxiliary. [17] , [20] Although diaryliodonium salts represent the most investigated class of hypervalent iodine(III) compounds in PET, there is scant patent literature [21] on how one might achieve the desired regiospecific radiofluorination based on the use of aryliodonium ylides (ArI=CX 2 ; X=electron-deficient substituent) as precursors with Meldrum’s acid auxiliaries. Here we report a spirocyclic hypervalent iodine(III)-mediated radiofluorination strategy, based on iodonium ylides ( Fig. 1b, 4 ), to afford 18 F-aryl fluorides in high radiochemical yields. The technique involves stable, easily purified precursors and is readily implemented with standard workup procedures. The conceptual advantages of excellent regioselectivity and viability of incorporation of 18 F into a wide array of non-activated (hetero)arenes make this methodology suitable for routine radiopharmaceutical production. Design of spirocyclic iodonium ylides for radiolabelling The initial goal of the present work was to discover an optimally designed auxiliary ( Fig. 1b, 4 ) capable of stabilizing the I(III) centre of the iodonium ylide precursors, particularly if bound to non-activated arenes, thereby disfavouring notorious I(III) decomposition [22] and disproportionation [23] pathways. As shown in Fig. 2a , the extent of such stabilization should still enable the formation of 18 F-labelled products via the addition/reductive elimination mechanism [16] , [24] that has been invoked for diaryliodonium salts and other I(III) species [15] , [16] , [17] , [20] , [25] , [26] . Initial experiments ( Fig. 2b ) with derivatives of Meldrum’s acid 9a and barbituric acid 8a , based on a challenging electron-neutral biphenyl substrate, provided radiochemical conversions of 47% and 53%, respectively. Analogues incorporating substituents on the nitrogen atoms of barbiturates 8b – d or alkyl groups other than methyl on the quaternary carbon of diesters 9b – d either exhibited poor stability at room temperature or were thick oils that were difficult to handle. These fruitless attempts led us to study a unique spirocyclic scaffold, which is rarely utilized in organic chemistry and has not been previously explored in radiochemistry. Gratifyingly, a spirocyclohexyl precursor, 10a , was a stable crystalline solid that showed reactivity towards 18 F-fluoride ion similar to that of 9a (52% incorporation yield). The well-tolerated initial reactions with 10a inspired us to modulate smaller spirocycles and we discovered that cyclobutyl 10b and cyclopentyl 10c groups led to significantly increased conversions, 70% and 85%, respectively ( Fig. 2b ; Supplementary Fig. 1 ). The biphenyl precursor 10c exhibited a significantly enhanced thermal stability over congeners incorporating alternative ligands under analogous radiolabelling conditions (DMF, 120 °C, 10 min). 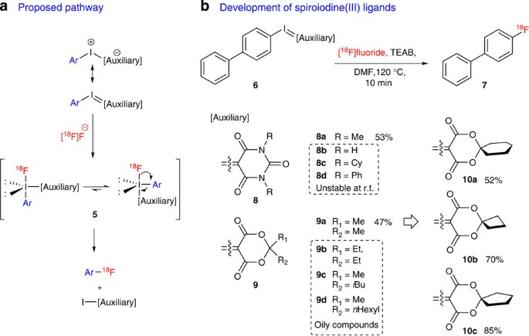Figure 2: Development of spirocyclic iodonium ylides for radiofluorination. (a) Proposed pathway. Radiofluorination of spiroiodonium ylides is proposed to occur through trigonal bipyramidal intermediate5. (b) Development and screening of spiroiodine(III) ligands. Conditions: biphenyl spiroiodine(III) precursor (2 mg), TEAB (7 mg), DMF (400 μl), 120 °C, 10 min. Incorporation yield and product identity were determined by radioTLC and radioHPLC, respectively (n=3). TEAB, tetraethylammonium bicarbonate; DMF,N,N-dimethylformamide. Figure 2: Development of spirocyclic iodonium ylides for radiofluorination. ( a ) Proposed pathway. Radiofluorination of spiroiodonium ylides is proposed to occur through trigonal bipyramidal intermediate 5 . ( b ) Development and screening of spiroiodine(III) ligands. Conditions: biphenyl spiroiodine(III) precursor (2 mg), TEAB (7 mg), DMF (400 μl), 120 °C, 10 min. Incorporation yield and product identity were determined by radioTLC and radioHPLC, respectively ( n =3). TEAB, tetraethylammonium bicarbonate; DMF, N , N -dimethylformamide. Full size image The labelling precursors 13 ( Fig. 3a ) were easily synthesized from the corresponding aryl iodine(III) derivatives 12 or by a one-pot procedure from aryl iodide 11 . These reactions were typically carried out under ‘open-flask’ conditions ( Supplementary Methods ) and in all cases afforded crystalline products. Among many commonly-used radiolabelling conditions, a simple combination of dried [ 18 F]fluoride with tetraethylammonium bicarbonate (TEAB [27] ) and spirocyclic iodine precursor in DMF was deemed to be optimal ( Supplementary Table 1 ). The use of 2,2,6,6-tetramethyl-1-piperidinyloxy and butylated hydroxytoluene, as radical scavengers, offered no improvement of radiolabelling efficiency. As shown in Fig. 3b , hindered alkyl substituents without activating groups were successfully radiolabelled with 18 F in 45–56% incorporation yield ( 15 and 16 , Supplementary Figs 2 and 3 ). Compound 15 represents a rare example of a highly sterically hindered 18 F-labelled benzene derivative bearing alkyl substituents. We next turned our attention to arenes with substituents at the benzyl position. Three substrates ( 17 – 19 ) underwent 18 F-incorporation in modest to good yields ( Supplementary Figs 4–6 ). A protected form of 4-[ 18 F]fluorobenzyl amine ( 18 )—an important building block—was prepared by the present method in 40% yield without the requirement of metal-mediated reduction from a nitrile precursor [28] , [29] . 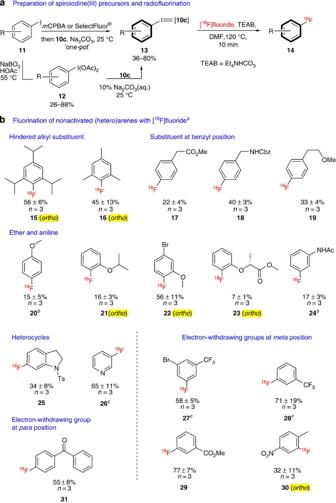Figure 3: Scope of spirocyclic hypervalent iodine(III)-mediated radiofluorination. (a) Preparation of spiroiodine(III) precursors and radiofluorination. (b) Fluorination of non-activated (hetero)arenes with [18F]fluoride.aRadiolabelling conditions: precursor (2 mg), TEAB (7 mg), DMF (400 μl), [18F]fluoride (1–3 mCi), 120 °C × 10 min. Incorporation yield was determined by radioTLC. The identity of labelled product was confirmed by radioHPLC.bReaction temperature 150 °C.cIncorporation yield was determined by radioHPLC. Non-activated arenes withorthofunctionalities are highlighted in yellow. TEAB, tetraethylammonium bicarbonate;mCPBA,meta-chloroperoxybenzoic acid. Figure 3: Scope of spirocyclic hypervalent iodine(III)-mediated radiofluorination. ( a ) Preparation of spiroiodine(III) precursors and radiofluorination. ( b ) Fluorination of non-activated (hetero)arenes with [ 18 F]fluoride. a Radiolabelling conditions: precursor (2 mg), TEAB (7 mg), DMF (400 μl), [ 18 F]fluoride (1–3 mCi), 120 °C × 10 min. Incorporation yield was determined by radioTLC. The identity of labelled product was confirmed by radioHPLC. b Reaction temperature 150 °C. c Incorporation yield was determined by radioHPLC. Non-activated arenes with ortho functionalities are highlighted in yellow. TEAB, tetraethylammonium bicarbonate; m CPBA, meta -chloroperoxybenzoic acid. Full size image Radiolabelling of non-activated and/or hindered arenes A range of other electron-rich arenes, the labelling of which constitutes an unmet need and a historical challenge, proved to be good substrates for the present 18 F-labelling strategy. This includes arenes incorporating alkoxy groups 20 – 23 , where 21 – 23 are concurrently challenged with hindered ortho substituents ( Supplementary Figs 7–10 ). Bromo derivative 22 represents a new building block that could be further functionalized or linked to complex molecular motifs through cross-coupling reactions [30] . Notably, a radiosynthesis of N -acetyl 3-[ 18 F]fluoroaniline ( 24 ) revealed an advantage over previous methods by avoiding the undesired formation of [ 18 F]fluoromethane generated via the reaction of [ 18 F]fluoride with a N , N , N -trimethylammonium-3-nitrobenzene triflate precursor [31] ( Supplementary Fig. 11 ). Indoline 25 and pyridine 26 were radiofluorinated in 34% and 65% incorporation yield, respectively, demonstrating the broad potential of our method for 18 F-labelling of nitrogen-containing heterocycles ( Supplementary Figs 12 and 13 ). Arenes displaying electron-withdrawing groups, including trifluoromethyl, halide, nitro and ester substituents at the meta (non-activated) positions ( Fig. 3b , 27 – 30 ), were also successfully radiofluorinated by the new protocol ( Supplementary Figs 14–17 ). Two arene substrates with the CF 3 pharmacophore ( 27 and 28 ) were successfully radiolabelled with 18 F at the meta -position in excess of 45% conversion. Compound 27 demonstrates compatibility with aryl halides and could be further functionalized via coupling reactions [30] . Ester 29 was labelled in 77% conversion and may be directly converted to 3-[ 18 F]fluorobenzyl alcohol, which is a key fragment of [ 18 F]lapatinib [32] . In the example of fluorobenzophenone 31 , we demonstrated that our method worked equally well for an activated arene with an electron-withdrawing group at the para position ( Supplementary Fig. 18 ). Few exceptions for this methodology are expected, which includes precursors with unprotected hydroxy groups, amines and carboxylic acids. The above-mentioned examples demonstrate that this radiofluorination technology is widely applicable in six major classes of arenes and overcomes the challenges in previous methodologies as well as offers unique building blocks that were previously inaccessible. Chromatographic analysis (radioTLC and radioHPLC) of crude reaction mixtures obtained in the course of this study showed that the sole radioactive products were the 18 F-radiolabelled arenes along with unreacted [ 18 F]fluoride. No other radioactive byproducts were detected. The unique selectivity can be, in part, explained by the substantial difference of electron densities between two carbon atoms attached to the I(III) center. A 13 C NMR study of our spirocyclic biphenyl based on 10c revealed that the ipso carbon ( Fig. 1, 4 ) resonates significantly downfield (114.3 p.p.m.) relative to the alpha carbon (57.2 p.p.m.) and is less shielded, indicating decreased electron density, and consequently greater propensity towards 18 F during reductive elimination. In contrast, diaryliodonium salts [22] do not exhibit a dramatic difference in 13 C chemical shifts, in accord with the reduced degree of regioselectivity in fluorination. Translation to PET radiopharmaceuticals To highlight the practical utility of spirocyclic hypervalent iodine(III)-based radiofluorination, we have demonstrated that established radiotracers that were previously accessible by [ 18 F]F 2 and known molecules with sensitive functionalities are well suited for labeling with [ 18 F]fluoride. As shown in Fig. 4 , a N,O -protected [ 18 F]fluorophenylalanine, 34 , was successfully labelled via the corresponding spiroiodine(III) precursor in 55% incorporation yield ( Supplementary Fig. 19 ). It is noteworthy that [ 18 F]fluorophenylalanine and its derivatives have only been synthesized via carrier-added [ 18 F]F 2 [33] , [34] , [35] or through cumbersome multi-step reactions starting with [ 18 F]fluoride culminating with chiral HPLC separations [36] . [ 18 F]Fluoroestrone ( 37 ), previously prepared by transition-metal-mediated methods [12] , [13] , was also synthesized, in 23% incorporation yield ( Supplementary Fig. 20 ). 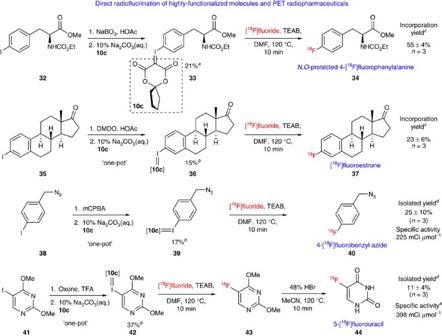Figure 4: Direct radiofluorination of highly functionalized molecules and PET radiopharmaceuticals. (a) Purified by recrystallization. (b) Purified by silica chromatography. (c) Incorporation yield and product identity were determined by radioTLC and radioHPLC, respectively (n=3). (d) Reported as uncorrected radiochemical yield and isolated by solid-phase extraction technique (n=3), radiochemical purity >95%. (e) Specific activity was determined based on intermediate43. DMDO, dimethyldioxirane; Oxone, potassium peroxysulphate; TFA, trifluoroacetic acid. Figure 4: Direct radiofluorination of highly functionalized molecules and PET radiopharmaceuticals. ( a ) Purified by recrystallization. ( b ) Purified by silica chromatography. ( c ) Incorporation yield and product identity were determined by radioTLC and radioHPLC, respectively ( n =3). ( d ) Reported as uncorrected radiochemical yield and isolated by solid-phase extraction technique ( n =3), radiochemical purity >95%. ( e ) Specific activity was determined based on intermediate 43 . DMDO, dimethyldioxirane; Oxone, potassium peroxysulphate; TFA, trifluoroacetic acid. Full size image Fluorine-18-labelled azides have found widespread use in ‘click’ syntheses of 18 F-labelled peptides [37] , [38] . For example, 4-[ 18 F]fluorobenzyl azide ( Fig. 4 , 40 ) is a common building block for such reactions that is synthesized by a lengthy four-step route [37] or via a diaryliodonium salt method using an esoteric flow device [39] . In the present work, we significantly improved and simplified the synthesis of 40 using a spiroiodine(III) precursor 39 , prepared from 4-iodobenzyl azide by a one-pot method, and directly radiolabelled and isolated 40 in 25% uncorrected radiochemical yield within 40 min, relative to dried [ 18 F]fluoride ( Supplementary Figs 21 and 22 and Supplementary Table 2 ). The methodology presented herein was also used to prepare a PET radiopharmaceutical, 5-[ 18 F]fluorouracil ( 44 ), which was difficult to achieve by S N Ar and was previously prepared by an electrophilic [ 18 F]F 2 method, that consequently results in low specific activity due to carrier F 2 (ref. 40 ). We converted 5-iodo-2,4-dimethoxypyrimidine to the corresponding spiroiodine(III) precursor 42 , which underwent a stepwise radiofluorination and deprotection by aqueous hydrobromic acid, to generate 44 in 11% isolated uncorrected radiochemical yield from dried [ 18 F]fluoride with a specific activity of 0.4 Ci μmol −1 ( Supplementary Figs. 23 and 24 & Supplementary Table 3 ), representing the radiosynthesis of 5-[ 18 F]fluorouracil from nucleophilic [ 18 F]fluoride for the first time. This reaction was carried out using ca . 300 mCi of starting [ 18 F]fluoride for proof of concept. We are presently scaling up and automating this reaction for clinical radiopharmaceutical production. Spiroiodine(III)-based precursors are stable species that have proven to enable direct and regioselective 18 F-labelling of non-activated and sterically hindered arenes with remarkably broad functional group compatibility. A wide range of non-activated arenes with structurally diverse and/or ortho functional groups, including esters, carbamates, halides, amides, nitro groups, trifluoromethyl groups, ketones and heterocycles, were efficiently radiolabelled by the developed method. Several 18 F-PET tracers and building blocks were successfully synthesized from [ 18 F]fluoride ion for the first time and/or the corresponding radiosyntheses were significantly simplified and improved via one-step reactions. Radiotracers prepared by this methodology were shown to be easily isolated in high radiochemical yields and specific acitivies, suitable for clinical translation. General methods for radioisotope production and preparation A GE PETtrace 16.5 MeV cyclotron was used for [ 18 F]fluoride production by the 18 O(p,n) 18 F nuclear reaction to irradiate 18 O-enriched water. [ 18 F]fluoride was delivered to a lead-shielded hot cell in 18 O-enriched water by nitrogen gas pressure. [ 18 F]fluoride was prepared for radiofluorination of aromatics by one of two methods: (A) A solution of base (for example, TEAB, 7 mg) in acetonitrile and water (1 ml, v/v 7:3) was added to an aliquot of target water (≤1 ml) containing the appropriate amount of [ 18 F]fluoride in a V-shaped vial sealed with a teflon-lined septum. The vial was heated to 110 °C while nitrogen gas was passed through a P 2 O 5 -Drierite column followed by the vented vial. When no liquid was visible in the vial, it was removed from heat, anhydrous acetonitrile (1 ml) was added and the heating was resumed until dryness. This step was repeated an additional three times. The vial was then cooled at room temperature under nitrogen pressure. The contents were resolubilized in the desired solvent (for example, DMF). (B) An aliquot of target water containing the appropriate amount of [ 18 F]fluoride was slowly passed through an anion exchange cartridge (MP1, ORTG, TN, USA), preactivated by flushing with NaHCO 3(aq) (8.4%, 1 ml) and water (2–3 ml, until neutral by a pH indicator). [ 18 F]fluoride was eluted using a solution of base (for example, TEAB, 7 mg) in acetonitrile and water (1 ml, v/v 7:3) into a V-shaped vial sealed with a teflon-lined septum. Drying and resolubilization were then performed as described above. For preparations involving crypt-222, drying was conducted at 95 °C. General methods for analysis of radiofluorination reactions Radioactivity was quantified using a Capintec Radioisotope Calibrator (CRC-712M) ion chamber. Radiochemical incorporation yields were determined by radioTLC. EMD TLC Silica gel 60 plates (10 × 2 cm 2 ) were spotted with an aliquot (1–5 μl) of crude reaction mixture ~1.5 cm from the bottom of the plate (baseline). Unless otherwise noted, TLC plates were developed in a chamber containing ethyl acetate until within 2 cm of the top of the plate (front). Analysis was performed using a Bioscan AR-2000 radio-TLC imaging scanner and WinScan software. Radiochemical identity and purity were determined by radioHPLC. A Phenomenex Luna C18, 250 × 4.6 mm, 5 μm HPLC column was used with a Waters 1515 Isocratic HPLC Pump equipped with a Waters 2487 Dual λ Absorbance Detector, a Bioscan Flow-Count equipped with a NaI crystal and Breeze software. Mobile phases and flowrates included 70% CH 3 CN, 30% 0.1 M NH 4 ·HCO 2(aq) , 1 ml min −1 ; 50% CH 3 CN, 50% 0.1 M NH 4 ·HCO 2(aq) , 1 ml min −1 , and 5% EtOH, 95% 0.1% AcOH (aq) , 1 ml min −1 . In order to account for immobilized radioactivity (which would not be accounted for by radioTLC), reaction vessels were decanted after quenching, and residual and solution radioactivity were separately quantified. In all cases, ≥95% of radioactivity remained in solution. General procedure for radiofluorination of arenes Azeotropically dried [ 18 F]Et 4 NF (typically 1–3 mCi, 37–110 MBq), resolubilized in DMF (400 μl), was added to a V-vial containing spiroiodine(III) precursor ( 13 , 2 mg). The reaction was heated at 120 °C for 10 min, and quenched with HPLC buffer (for example, 60:40 CH 3 CN:H 2 O+0.1 N ammonium formate, 1 ml). Fluorine incorporation and product identities were determined by radioTLC and radioHPLC ( n ≥3). For radioTLC and radioHPLC data, see Supplementary Figs 1–22 . Conditions were optimized for radiofluorination of 10c to produce [ 18 F]7 . Radiofluorination of all other substrates was performed under identical conditions and they remained unoptimized. For certain products that were detected in low yield (that is, 20 , 24 ), a reaction temperature of 150 °C proved superior to the general procedure temperature of 120 °C. Specific activity of isolated radioactive products Specific activity was determined by measurement of the UV absorbance of a known amount of radioactivity under identical analytical HPLC conditions used to generate a calibration curve for the corresponding nonradioactive standard. See Supplementary Figs 22 and 24 , and Supplementary Tables 2 and 3 for details. General procedure for synthesis of iodonium ylides To a solution of the auxiliary acid ( 8 – 10 , 0.25 mmol) in 10% Na 2 CO 3(aq) (w/v, 0.75 ml, 0.33 M solution) was added ethanol (1 ml) followed quickly by diacetoxyiodoarene ( 11 , 0.25 mmol). The reaction mixture was vigorously stirred at room temperature for 0.5–4 h, until full conversion of starting materials was determined by TLC. The reaction mixture was then diluted with water (~8 ml), and extracted with DCM (3 × 10 ml). The combined organic extracts were dried with anhydrous Na 2 SO 4 , filtered and concentrated. To the residue was added ethyl acetate and hexanes to induce precipitation (at room temperature or –25 °C). Solids were collected by filtration and purified by flash chromatography if necessary. For 1 H, 13 C and 19 F spectra of new compounds, see Supplementary Figs 25–118 . How to cite this article: Rotstein, B. H. et al. Spirocyclic hypervalent iodine(III)-mediated radiofluorination of non-activated and hindered aromatics. Nat. Commun. 5:4365 doi: 10.1038/ncomms5365 (2014).